Edge and confinement effects allowin situmeasurement of size and thickness of liquid-exfoliated nanosheets Two-dimensional nanomaterials such as MoS 2 are of great interest both because of their novel physical properties and their applications potential. Liquid exfoliation, an important production method, is limited by our inability to quickly and easily measure nanosheet size, thickness or concentration. Here we demonstrate a method to simultaneously determine mean values of these properties from an optical extinction spectrum measured on a liquid dispersion of MoS 2 nanosheets. The concentration measurement is based on the size-independence of the low-wavelength extinction coefficient, while the size and thickness measurements rely on the effect of edges and quantum confinement on the optical spectra. The resultant controllability of concentration, size and thickness facilitates the preparation of dispersions with pre-determined properties such as high monolayer-content, leading to first measurement of A-exciton MoS 2 luminescence in liquid suspensions. These techniques are general and can be applied to a range of two-dimensional materials including WS 2 , MoSe 2 and WSe 2 . Over the last few years the study of two-dimensional (2D) nanomaterials has become an important area of nanoscience [1] , [2] , [3] , [4] . The palette of 2D materials currently under study has expanded from graphene [3] , [5] , to include transition metal dichalcogenides (TMDs) such as MoS 2 and WSe 2 , layered transition metal oxides such as MnO 2 and TiTaO 5 and a host of other interesting structures such as GaS, germanane and Bi 2 Te 3 (refs 1 , 2 , 4 , 6 ) These materials are diverse, including metals, semiconductors, insulators or superconductors [1] , [4] , [7] , and display a range of interesting properties from thickness-dependent bandgaps [4] to catalytic activity [1] . These properties make them useful for both fundamental studies and applications in areas as diverse as optoelectronics, electrochemistry and medicine. While 2D materials can be grown directly [8] , they are generally obtained by exfoliation of layered crystals. This has long been possible by mechanical exfoliation, leading to samples of very high quality, but at very low throughput [9] , [10] , [11] . When larger production rates are required, chemical methods [12] , [13] , [14] , [15] , often based on ion intercalation, have been used to exfoliate layered crystals in liquids [2] . However, even though these methods result in large quantities of monolayers, they are time consuming, involving harsh chemical treatments, which must be carried out in an inert atmosphere. More recently, a much simpler method, liquid phase exfoliation (LPE), has been reported [16] , [17] , [18] , [19] , [20] , [21] , [22] , [23] , [24] , [25] , [26] , [27] . This method involves the sonication [18] or shearing [27] of layered crystals in certain solvents or solutions of surfactants or polymers. It results in the exfoliation of the layered crystal to give large numbers of 2D nanosheets, which are stabilized by interaction with the liquid. The resultant dispersions can be easily processed into films, coatings or composites: systems which are ideal for applications in a range of areas from batteries [28] , [29] to photodetectors [30] to reinforced materials. [21] , [25] , [31] This method is general and has been used to give exfoliated dispersions of graphene [16] , [17] , [20] , BN, [18] , [23] , [25] TMDs such as MoS 2 and WS 2 [18] , [19] , [24] , [26] , [29] , [32] , transition metal oxides such as MnO 2 (ref. 29 ) and MoO 3 (ref. 33 ), as well as more exotic structures such as Ti 3 C 2 F 2 nanosheets [34] or functionalized-layered double hydroxides [35] . In fact, we expect this method to be applicable to any layered compound, where the layers are bound predominately by van der Waals interactions. While LPE is a versatile and useful technique, it has some notable disadvantages. First, optical characterization of nanosheet dispersions is hampered by the presence of a scattering background, which depends sensitively on the size of the dispersed nanosheets [18] , [24] . As such, it is not clear how to define an intrinsic extinction coefficient, making even concentration measurements challenging. Moreover, LPE gives nanosheets, which are polydisperse both in thickness and lateral size. While lateral size separation is possible [24] , [36] , separation by thickness is more challenging. In addition, measurement of nanosheet size is tedious, requiring time-consuming statistical microscopic analysis. While approximate in situ measurements of lateral size can be made optically [37] , no in situ method for nanosheet thickness measurement exists. To measure thickness, it is necessary to deposit nanosheets on surfaces, avoiding aggregation and use statistical Raman or atomic force microscopy (AFM) [38] . This can be very time consuming if a mean over many nanosheets is required. Ultimately, a simple method to separate nanosheets by size and thickness would be very useful. More importantly, a fast in situ method to measure both lateral size and thickness of nanosheets is urgently required. Here we address these points. We demonstrate size-selection techniques which give fractions with optical extinction spectra which vary systematically with both nanosheet size and thickness. By combining the spectroscopic analysis with statistical microscopic analysis, we generate quantitative relationships between spectral properties and nanosheet dimensions. Quantifying these effects allows an extinction spectrum to be used to obtain not only the nanosheet concentration but also the nanosheet length and thickness. The ability to control size and thickness is very useful, facilitating for example the preparation of monolayer-rich dispersions. Critically, we find this methodology to be general to a range of 2D materials. Size selection of MoS 2 nanosheets To produce dispersions of MoS 2 nanosheets with varying thickness and lateral size distributions from the same stock sample, we used a simple centrifugation technique based on band sedimentation (BS, Fig. 1a ). A stock dispersion of the surfactant-exfoliated [29] nanomaterial was layered on top of a race layer of higher density and subjected to a short (typically 10–40 min) centrifugation using a normal benchtop centrifuge. The centrifugation leads to the spreading of the material through the vial such that nanosheet mass increases going from top to bottom [39] . Fractionation then allows the collection of size-selected samples. Similar techniques have previously been described in literature to sort carbon nanotubes [40] , [41] , graphene oxide nanosheets [42] and nanoparticles [43] by their lateral dimensions. While the higher density of the race layer is normally achieved using a density gradient medium, we use a combination of water and deuterated water to minimize the additive content and avoid potential interactions between gradient medium and MoS 2 . 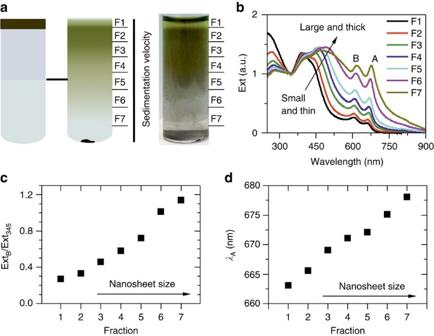Figure 1: MoS2band sedimentation and size-dependent extinction spectra. (a) Experimental setup for band sedimentation centrifugation involving layering a nanomaterial stock dispersion on top of a race layer. Centrifugation leads to spreading of the material throughout the vial and separation of the nanosheets according to their sedimentation velocities and so their size. Fractions as indicated are withdrawn from top to bottom. (b) Extinction spectra of the fractions normalized to the local minimum at 345 nm. The positions of the A- and B-excitons are marked. (c) Ratio of extinction at B-exciton to that at 345 nm, ExtB/Ext345plotted versus fraction number. (d) Peak position (wavelength) of the A-exciton,λA, as a function of fraction number. We propose thatλAand ExtB/Ext345can be used as metrics for flake thickness and length, respectively. Figure 1: MoS 2 band sedimentation and size-dependent extinction spectra. ( a ) Experimental setup for band sedimentation centrifugation involving layering a nanomaterial stock dispersion on top of a race layer. Centrifugation leads to spreading of the material throughout the vial and separation of the nanosheets according to their sedimentation velocities and so their size. Fractions as indicated are withdrawn from top to bottom. ( b ) Extinction spectra of the fractions normalized to the local minimum at 345 nm. The positions of the A- and B-excitons are marked. ( c ) Ratio of extinction at B-exciton to that at 345 nm, Ext B /Ext 345 plotted versus fraction number. ( d ) Peak position (wavelength) of the A-exciton, λ A , as a function of fraction number. We propose that λ A and Ext B /Ext 345 can be used as metrics for flake thickness and length, respectively. Full size image After the BS centrifugation, ~6 mm deep fractions were collected from the vial, where the smallest, slowest sedimenting species are found in the top fraction (F1). We measured extinction spectra for each fraction. To distinguish it from the true absorbance, Abs, we will refer to the extinction as Ext, where T =10 −Ext ( T is the optical transmittance). The normalized extinction spectra of a typical set of fractions ( Fig. 1b ) display the excitonic transitions typical of MoS 2 (ref. 7 ). However, we find that they show very distinct and clear changes that obviously reflect the different size distributions of the MoS 2 nanosheets in the dispersion ( Supplementary Fig. 1 ). The extinction-weighted sum of the individual extinction spectra of the fractions matched well to the stock dispersion ( Supplementary Fig. 2 ) confirming that the changes in the extinction spectra indeed reflect the separation process. In Figure 1b , we see very pronounced spectral changes from fraction to fraction. These changes were quantified by plotting the ratio of extinction at the B-exciton peak (605 nm) to that at the local minimum at 345 nm, Ext B /Ext 345 ( Fig. 1c ). We observe a considerable change with a fourfold increase in this ratio occurring from F1 to F7. Since no such observation has been made when exploring the extinction spectra of films of restacked chemically exfoliated MoS 2 of different nanosheet thicknesses [14] , this strongly suggests that the spectral changes shown in Fig. 1b,c are related to changes in nanosheet lateral size. This implies that the extinction spectra contain quantitative information on the lateral dimensions of the nanosheets. In addition to the obvious spectral changes, it is clear that the position of the A-exciton, λ A , varied from fraction to fraction. Because the extinction spectra for MoS 2 dispersions include a contribution from a size-dependent scattering background [18] , we found λ A using the second derivative of the extinction spectra ( Supplementary Fig. 3 ). The resultant peak position is plotted in Fig. 1d , showing a clear trend versus fraction number ( Fig. 1d ). This is consistent with red-shifting of the peak for thicker nanosheets (that is, in higher fractions) such that λ A increases as the number of layers per nanosheet, N , increases. Such behaviour has been observed for a number of TMDs and is due to confinement effects [14] , [44] , [45] . This implies that, in addition to lateral size information, the extinction spectra contain quantitative information on the thickness of the nanosheets. Differentiating absorbance from scattering However, before any quantitative information can be extracted from the extinction spectra, it is important to realize that such spectra include contributions from both absorbance and scattering. In fact, scattering is known to be significant for dispersions of nanosheets [18] , especially those with large lateral size [24] . To assess the effects of scattering, we prepared a set of MoS 2 dispersions with a range of flake sizes. The concentration was measured by filtration and weighing to allow the calculation of extinction (as well as absorption and scattering) coefficients ( Supplementary Fig. 4 ). Extinction spectra were measured and converted to extinction coefficient ( ε ) spectra as shown in Fig. 2a (N.B. Ext= εCl , where C is the concentration and l is the cell length). We used an integrating sphere to differentiate the contributions of absorbance and scattering, leading to the absorption ( α ) and scattering ( σ ) coefficient spectra shown in Fig. 2b,c (N.B. ε ( λ )= α ( λ )+ σ ( λ )). It is clear from these spectra that scattering makes a significant contribution to the extinction spectra. For λ >700 nm, σ ∝ λ − n , with n roughly in the range 1–4 as suggested previously [18] , [24] , [46] . However, for λ <700 nm, σ ( λ ) is broadly similar in shape to α ( λ ). This is important because, as a result, α ( λ ) and ε ( λ ) are also similar in shape. This means that any metrics extracted from an extinction spectrum will reflect the information contained in the absorption spectrum. To test this, we extracted λ A from both extinction and absorbance spectra, plotting one versus another for a range of fractions as shown in Fig. 2d . We also plotted Ext B /Ext 345 versus Abs B /Abs 345 in Fig. 2e . For all but the largest fractions (that is, F6 and F7), we find good scaling between the values extracted from extinction and absorption spectra. This indicates that, even though scattering is always present, information encoded in an absorption spectrum can be effectively extracted from the extinction spectrum. 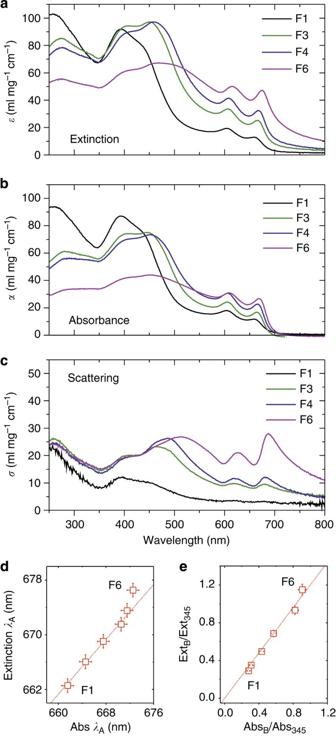Figure 2: Extinction, absorbance and scattering spectra. (a) Wavelength dependence of optical extinction coefficient,ε, for fractions F1, F3, F4 and F6. NBεis defined byT=10−εClwhereTis the transmittance,Cis the MoS2concentration andlthe cell length.εcan be split into contributions from absorption,α, and scattering,σ, such thatε=α+σ. (b,c) Wavelength dependence of (b) optical absorption coefficient,α, and (c) optical scattering coefficient,σ. (d) A-exciton position measured from the extinction spectra (Fig. 2a) plotted versus that measured from the absorption spectra (Fig. 2b) for fractions F1–F6. (e) ExtB/Ext345(measured from the extinction spectra,Fig. 2a) plotted versus AbsB/Abs345(measured from the absorption spectra,Fig. 2b) for fractions F1–F6. Figure 2: Extinction, absorbance and scattering spectra. ( a ) Wavelength dependence of optical extinction coefficient, ε , for fractions F1, F3, F4 and F6. NB ε is defined by T =10 − εCl where T is the transmittance, C is the MoS 2 concentration and l the cell length. ε can be split into contributions from absorption, α , and scattering, σ , such that ε = α + σ . ( b , c ) Wavelength dependence of ( b ) optical absorption coefficient, α , and ( c ) optical scattering coefficient, σ . ( d ) A-exciton position measured from the extinction spectra ( Fig. 2a ) plotted versus that measured from the absorption spectra ( Fig. 2b ) for fractions F1–F6. ( e ) Ext B /Ext 345 (measured from the extinction spectra, Fig. 2a ) plotted versus Abs B /Abs 345 (measured from the absorption spectra, Fig. 2b ) for fractions F1–F6. Full size image The effect of nanosheet length on optical spectra To test whether the extinction spectrum contains useful information about nanosheet length, we characterized a number of fractions using transmission electron microscopy (TEM). Representative TEM images of dispersions which are expected to contain large and small nanosheets are depicted in Fig. 3a–d . These images clearly show the expected size differences. To quantify these effects, we performed statistical analysis of nanosheet lengths for both band-sedimented dispersions and dispersions prepared by conventional centrifugation at different rates ( Supplementary Figs 5–7 ). We note that BS has the clear advantage of producing much narrower distributions ( Supplementary Fig. 7 ). However, homogenous centrifugation results in larger volumes and so larger quantities of separated materials. We found that the fractions described above contained nanosheets with mean lengths which varied from ~60 (F1) to 360 nm (F6), although considerably larger flakes (mean length up to 600 nm) can be made by adjusting BS conditions (that is, centrifuging at 2k r.p.m., 10 min). 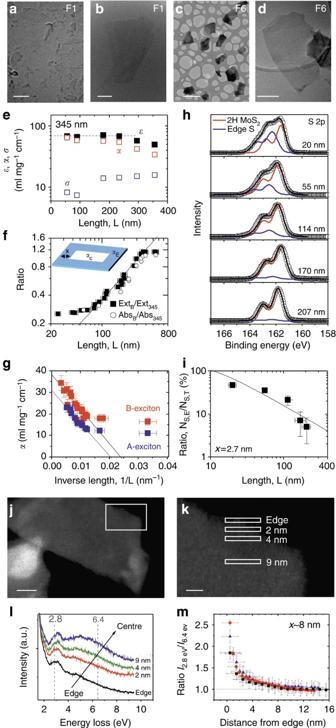Figure 3: Length metric and edge effects. (a,b) Representative TEM images of slowly sedimenting MoS2nanosheets (small flakes, F1, (a) scale bar, 100 nm, (b) scale bar, 10 nm). (c,d) Representative TEM images of faster sedimenting MoS2nanosheets (large flakes, F6, (c) scale bar, 1 μm, (d) scale bar, 100 nm). (e) Extinction (ε), absorption (α) and scattering (σ) coefficients at 345 nm plotted versus nanosheet length. The line represents ‹ε›=69 ml mg−1cm−1. (f) Ratio of extinction at B-exciton to that at 345 nm, ExtB/Ext345, plotted versus the lateral dimensions of the flake (expressed as mean length,L, obtained by statistical TEM analysis). The line is a fit to equation (4). Also shown is the equivalent data taken from the absorbance spectra (AbsB/Abs345). The inset schematically shows the division of a nanosheet into edge and central regions. (g) Absorption coefficient,α, at both A- and B-excitons plotted versus inverse nanosheet length. The dashed lines are fits to equation (1). (h) Fitted XPS S2p core-level spectra of filtered MoS2dispersions with different mean flake lengths. The additional component at higher binding energies is attributed to edgeS. (i) Fraction of S2p signal associated with edgeSas a function of flake length. This fraction is equal to the ratio of edgeSto totalSatoms. The line represents a fit to equation (2) and yields the width of the edge region to bex=2.7±0.5 nm. (j) Scanning transmission electron microscopy (STEM) image of MoS2nanosheets (scale bar, 20 nm). (k) STEM image of the region marked by the box injshowing the edge region of a typical MoS2nanosheet (scale bar, 5 nm). The boxes indicate the regions over which EEL spectra were acquired and analyzed. (l) Summed EEL spectra, normalized to the zero-loss peak, of the regions marked by the boxes ink(same data set asSupplementary Fig. S12c). The EEL spectra exhibited gradual changes when moving from the edge to the centre. (m) Plot of EELS intensity ratio at 2.8 eV to that at 6.4 eV (as indicated inl) as a function of distance from the edge. Data from three different regions are shown. The intensity ratio saturates at ~8 nm from the edge. Figure 3: Length metric and edge effects. ( a , b ) Representative TEM images of slowly sedimenting MoS 2 nanosheets (small flakes, F1, ( a ) scale bar, 100 nm, (b) scale bar, 10 nm). ( c , d ) Representative TEM images of faster sedimenting MoS 2 nanosheets (large flakes, F6, ( c ) scale bar, 1 μm, ( d ) scale bar, 100 nm). ( e ) Extinction ( ε ), absorption ( α ) and scattering ( σ ) coefficients at 345 nm plotted versus nanosheet length. The line represents ‹ ε ›=69 ml mg −1 cm −1 . ( f ) Ratio of extinction at B-exciton to that at 345 nm, Ext B /Ext 345 , plotted versus the lateral dimensions of the flake (expressed as mean length, L , obtained by statistical TEM analysis). The line is a fit to equation (4). Also shown is the equivalent data taken from the absorbance spectra (Abs B /Abs 345 ). The inset schematically shows the division of a nanosheet into edge and central regions. ( g ) Absorption coefficient, α , at both A- and B-excitons plotted versus inverse nanosheet length. The dashed lines are fits to equation (1). ( h ) Fitted XPS S2p core-level spectra of filtered MoS 2 dispersions with different mean flake lengths. The additional component at higher binding energies is attributed to edge S . ( i ) Fraction of S2p signal associated with edge S as a function of flake length. This fraction is equal to the ratio of edge S to total S atoms. The line represents a fit to equation (2) and yields the width of the edge region to be x =2.7±0.5 nm. ( j ) Scanning transmission electron microscopy (STEM) image of MoS 2 nanosheets (scale bar, 20 nm). ( k ) STEM image of the region marked by the box in j showing the edge region of a typical MoS 2 nanosheet (scale bar, 5 nm). The boxes indicate the regions over which EEL spectra were acquired and analyzed. ( l ) Summed EEL spectra, normalized to the zero-loss peak, of the regions marked by the boxes in k (same data set as Supplementary Fig. S12c ). The EEL spectra exhibited gradual changes when moving from the edge to the centre. ( m ) Plot of EELS intensity ratio at 2.8 eV to that at 6.4 eV (as indicated in l ) as a function of distance from the edge. Data from three different regions are shown. The intensity ratio saturates at ~8 nm from the edge. Full size image Before discussing the possibility of developing a length metric, it is worth investigating how the extinction, absorbance and scattering coefficients depend on nanosheet length. Interestingly, the data in Fig. 2a suggests that when λ =345 nm, ε is relatively invariant with fraction number and so with L . In Fig. 3e , we plot ε , α and σ (all at λ =345 nm) versus L . We find ε at λ =345 nm to be dominated by absorption and to be invariant with length with a mean of ‹ ε ›≈69 ml mg −1 cm −1 ( Supplementary Fig. 8 ). This allows extinction spectra to be used to estimate the nanosheet concentration for dispersions of any flake length (for L <300 nm at least). Previously, this was not possible because the influence of the size-dependent scattering background was unknown [18] , [24] . To assess the possibility of using Ext B /Ext 345 as a metric for length, we plot this parameter versus mean nanosheet length, L , for a range of size-selected dispersions in Fig. 3f . We see a clear increase in Ext B /Ext 345 with increasing L , indicating that this ratio can be used as a metric for L . The ratio Abs B /Abs 345 , calculated from the true absorbance spectra follows the same trend in line with the data in Fig. 2e . We propose that these size-dependent spectral changes reflect the effect of flake edges on the local electronic structure, density of states and hence local optical absorption coefficient of the nanosheets [47] . This effect may be due to structural relaxations or the misalignment of stacked monolayer edges. In any case, the observed absorption spectrum will be the sum of edge and centre contributions. Because the population ratio of edge to centre atoms increases with decreasing nanosheet size, we expect the spectral shape to be size dependent. We can model this behaviour by treating the flakes as consisting of edge (E) and centre (C) regions ( Fig. 3f inset), each of which has a well-defined absorption coefficient (that is, α E and α C ). Modelling the nanosheets as arbitrary 2D shapes with long dimension, L , and aspect ratio, k ( k =length/width, Supplementary Note 1 ), we can take the area-weighted sum of centre and edge absorption coefficients to derive an expression for the average effective nanosheet extinction coefficient: where Δ α = α E − α C and x is the width of the edge region. To test this, we plot the absorbance coefficient at both the A- and B-exciton versus the inverse nanosheet length in Fig. 3g . We observed good linearity as predicted by equation (1) so long as L >60 nm, below which saturation occurs, consistent with small-flake absorbance being dominated by edges. The fit implies values of α C of 31±1 and 38±2 ml mg −1 cm −1 for the A- and B-excitons, respectively, while saturation implies equivalent values for α E of 11±1 and 17±1 ml mg −1 cm −1 . Because TEM analysis shows k ≈2 for all nanosheet lengths ( Supplementary Fig. 5 ), we can use the fits, coupled with equation (1), to estimate x =12±7 nm. This value is larger than would be expected for effects solely due to electronic edge states, suggesting more complex phenomena to be at work. However, it is worth noting that scanning tunnelling microscopy measurements on MoS 2 on graphite have shown a distinct edge region at least 5 nm thick [48] . Nevertheless, the effects described here may not be universal but perhaps specific to nanosheets surrounded by a weakly interacting environment (for example, surfactant micelle or solvent solvation shell). To confirm the presence of a distinct edge region, X-ray photoelectron spectroscopy (XPS) was performed on a range of films prepared from nanosheets of different sizes. No systematic changes in the Mo core-level spectra ( Supplementary Fig. 9 ) were detected. However, in addition to the expected 2H component of the S2p core-level spectra, as long as we investigate freshly prepared samples, we observe an extra component that cannot be identified with known morphologies, for example 1 T MoS 2 ( Fig. 3h ) (also Supplementary Fig. 10 ). Critically, the intensity of this additional component increases with decreasing flake length allowing us to associate it with the edge region. Then, the fraction of the S2p signal associated with this component will equal the fraction of S atoms associated with the edge region; N S,E / N S,T . This ratio is plotted as a function of flake length in Fig. 3i . The fraction of S atoms within a distance x from the edge is given by This expression describes the data in Fig. 3i rather well, giving a value of x =2.7±0.5 nm. We note that this value for x is lower than the one quoted above, suggesting that XPS probes edge properties which are distinct to those seen by absorbance measurements. To further illustrate differences in electronic structure between edge and centre of MoS 2 nanosheets, we have performed scanning TEM (STEM) imaging ( Fig. 3j–k ) and low-loss STEM electron energy-loss spectroscopy (EELS, Supplementary Figs 11 and 12 ). Moving inward from the nanosheet edge ( Fig. 3k ), the EEL spectra ( Fig. 3l ) exhibited gradual changes in the energy-loss regions between 2 and 10 eV. These changes reflect differences in electronic structure near the flake edge compared with the centre. We examined these changes via the ratio of EELS intensities at two energies, for example, 2.8 and 6.4 eV, I 2.8 eV / I 6.4 eV . These specific positions were chosen, as they show the largest changes in the spectra with distance from the edge. We have calculated this ratio for a number of spectra, measured at a range of positions on three different nanosheets, as a function of distance from nanosheet edge as shown in Fig. 3m . We took care to choose regions of uniform thickness to exclude effects from thickness variations in the EELS. This data clearly shows I 2.8 eV / I 6.4 eV to fall off with increasing distance from the edge before saturating for spectra collected at a distance of >8 nm from the flake edge. This suggests the presence of a distinct edge region with thickness of x ~8 nm in good agreement with the optical measurements (taking into account limitations to the spatial resolution). However, this result has to be interpreted with caution, since in this region of the low-loss spectra the exact origin of the peaks remains uncertain. The strong effect of nanosheet edges on electronic properties is also consistent with recent reports, which show MoS 2 in the vicinity of edges [48] , [49] or grain boundaries [50] to have electronic properties distinct from the central regions. Incidentally, this suggests that this approach could be used to measure grain size in chemical vapour deposition-grown MoS 2 . Length metric based on nanosheet edge effects We can use our model to understand the size-dependent changes to the shape of absorption spectra. We represent the spectral shape by the ratio of absorbance intensities at two distinct wavelengths, λ 1 and λ 2 . Using equation (1), we can express this as Because of the linear relationship between Ext B /Ext 345 and Abs B /Abs 345 ( Fig. 2e ), we can re-write this as Equation (4) can be used to fit the data in Fig. 3f , showing very good agreement, at least in the size range of 70–350 nm. Once the fit parameters are known, equation (4) can be rearranged to give a quantitative relationship between L and Ext B /Ext 345 : By assessing the root-mean-square relative difference between data and fit we estimate the error in L to be <10%. This is important and it allows Ext B /Ext 345 to be used to assess flake length for MoS 2 suspended in liquids simply by measuring the extinction spectrum. It works effectively for nanosheets in the size range 70< L <350 nm, which is almost exactly the range of nanosheets typically produced by LPE. For larger nanosheets, a different metric, based on the scattering exponent n can be used ( Supplementary Figs 13–16 and Supplementary Note 2 ). Nanosheet thickness metric based on confinement effects While a spectroscopic method to determine nanosheet length is undoubtedly important, even more useful would be an in situ method to assess thickness. As discussed above, it is clear that the position of the A-exciton peak in the absorbance spectrum has the potential to provide such a metric [14] , [44] . However, the number of layers per flake, N , must be measured before the relationship between peak position and N can be quantified. To do this, we deposited nanosheets from a number of fractions onto Si/SiO 2 wafers for characterization by AFM ( Fig. 4a,b ). In this way, we measured mean thicknesses for a large number of nanosheets across a number of fractions ( Fig. 4c and Supplementary Figs 17–19 ). 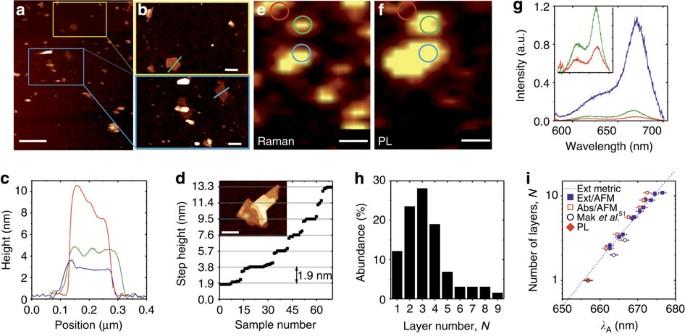Figure 4: Thickness metric. (a) Representative overview AFM images of a surfactant-exfoliated MoS2dispersion deposited on Si/SiO2wafers (scale bar, 1 μm). (b) Zoomed-in AFM images of the regions indicated ina. (c) Height profiles of the nanosheets in (b). (d) Heights of steps observed on deposited MoS2nanosheets such as that displayed in the inset (scale bar, 250 nm). The step height is found to be a multiple of 1.9 nm. (e) Raman (integrated A1gphonon area, scale bar, 1 μm) and (f) PL maps (excitation 532 nm, integrated area from 640–700 nm, scale bar 1 μm) of the region shown ina. (g) Photoluminescence spectra of the areas marked by circles (colour coded). The blue circle and spectrum, respectively, is associated with a flake of apparent height 3 nm (Fig. 4c). Inset: zoom-in of PL from multi-layered flakes marked by red and green circles associated with flakes of apparent thickness 5–7 nm (Fig. 4c). (h) Example (fraction F2) of a layer number histogram after conversion of AFM height to number of layers. (i) Plot of the mean number of layers as obtained from AFM thickness analysis versus the wavelength associated with the A-exciton measured from both extinction and absorbance spectra. The vertical error bars represent the standard error of the AFM height distribution. The red filled diamond represents free-standing micromechanically cleaved MoS2monolayer, whereλAwas obtained from the PL peak position. The experimental findings are consistent with literature data on the photoluminescence of free-standing MoS2extracted from Maket al.51NB profiles incare colour coded with the lines inb. Figure 4: Thickness metric. ( a ) Representative overview AFM images of a surfactant-exfoliated MoS 2 dispersion deposited on Si/SiO 2 wafers (scale bar, 1 μm). ( b ) Zoomed-in AFM images of the regions indicated in a . ( c ) Height profiles of the nanosheets in ( b ). ( d ) Heights of steps observed on deposited MoS 2 nanosheets such as that displayed in the inset (scale bar, 250 nm). The step height is found to be a multiple of 1.9 nm. ( e ) Raman (integrated A 1g phonon area, scale bar, 1 μm) and ( f ) PL maps (excitation 532 nm, integrated area from 640–700 nm, scale bar 1 μm) of the region shown in a . ( g ) Photoluminescence spectra of the areas marked by circles (colour coded). The blue circle and spectrum, respectively, is associated with a flake of apparent height 3 nm ( Fig. 4c ). Inset: zoom-in of PL from multi-layered flakes marked by red and green circles associated with flakes of apparent thickness 5–7 nm ( Fig. 4c ). ( h ) Example (fraction F2) of a layer number histogram after conversion of AFM height to number of layers. ( i ) Plot of the mean number of layers as obtained from AFM thickness analysis versus the wavelength associated with the A-exciton measured from both extinction and absorbance spectra. The vertical error bars represent the standard error of the AFM height distribution. The red filled diamond represents free-standing micromechanically cleaved MoS 2 monolayer, where λ A was obtained from the PL peak position. The experimental findings are consistent with literature data on the photoluminescence of free-standing MoS 2 extracted from Mak et al. [51] NB profiles in c are colour coded with the lines in b . Full size image However, conversion of the measured height into the actual number of monolayers per flake, N , is challenging due to adsorbed surfactant on both flakes and substrate. This means both surfactant-tip and surface-tip interactions contribute to the apparent height of the nanosheets, making N assessment difficult. To resolve this, we utilized the fact that incompletely exfoliated nanosheets often display terraces separated by steps associated with flake edges ( Fig. 4d inset). By analyzing the apparent AFM height on a large number of steps over many flakes [27] and plotting the step height in ascending order ( Fig. 4d ), it is clear that the step height is always a multiple of 1.9 nm. Even though this is larger than expected for monolayer MoS 2 , the absence of smaller step heights implies surfactant-exfoliated MoS 2 to display apparent monolayer heights of 1.9 nm (cf 1.1 nm for chemically exfoliated MoS 2 ) [14] . Furthermore, the thinnest flakes we have observed have an apparent height of 3 nm, consistent with a monolayer height of 1.9 nm plus ~1 nm surfactant under the flakes Unequivocal evidence that the nanosheets with an apparent height of 3 nm are monolayered MoS 2 can be obtained using photoluminescence (PL) and Raman spectroscopy, which allows identification of mono-, bi- and tri-layer MoS 2 (refs 38 , 44 ). For this, we relocated the sample area characterized by AFM ( Fig. 4a,b ) to a Raman microscope to optically characterize those flakes with known AFM thickness. Raman mapping, plotted as intensity of the A 1g mode in Fig. 4e , shows the presence of many MoS 2 flakes on the substrate in these regions. Critically, some of these flakes also display PL ( Fig. 4f ). The observed PL (and Raman spectra) from flakes with a height of ~3 nm was always consistent with monolayered MoS 2 ( Fig. 4c,g and Supplementary Figs 20–22 ). In contrast, slightly thicker flakes (for example, 5–7 nm in height), showed weaker PL with a clear shoulder at 620 nm, consistent with bi- and few-layered species [38] , [51] , [52] , [53] . This combination of AFM, Raman and PL spectroscopy clearly shows that surfactant-exfoliated monolayers display an apparent height of 3 nm with every additional monolayer contributing an extra 1.9 nm. This in turn allows the conversion of the mean AFM height obtained by statistical analysis of a given dispersion drop-cast on Si/SiO 2 wafers to the actual number of layers. This is depicted in Fig. 4h for a BS fraction, which optical measurement showed to have a low mean nanosheet thickness (that is, F2 with A-exciton position 666 nm≡1.86 eV). These results allow us to use AFM to measure the mean value of N in different fractions and so quantify the relationship between the mean number of monolayers per nanosheet, N , and the measured A-exciton position, λ A . We plot this data in Fig 4i for λ A taken both from extinction and absorption spectra. In both cases, the data are very similar, showing a well-defined relationship between N and λ A . The data point for the monolayer was obtained from determining the A-exciton energy from the PL of free-standing micromechanically cleaved MoS 2 ( Supplementary Fig. 23 , in absence of surfactant). We can test these results by comparing them to literature data [51] for A-exciton position for mono-, bi- and tri-layer mechanically exfoliated MoS 2 , finding very close agreement. This suggests any solvatochromic effect [54] associated with the presence of adsorbed sodium cholate to be small as confirmed by additional experiments ( Supplementary Fig. 24 ). The data in Fig. 4i clearly show an exponential relationship between N and λ A . Fitting the data where λ A is taken from the extinction spectrum gives with λ A in nanometre. This expression can be used to find the mean number of monolayers per nanosheet directly from the extinction spectrum of a MoS 2 dispersion. However, we note that for N ~10, the extinction and absorbance data begin to diverge, as scattering becomes more important. Thus, while equation (5) is only accurate for N <10, this is not a serious limitation as LPE typically gives dispersions with N <10. In addition, because the properties of MoS 2 become bulk like as N approaches 10 (refs 38 ), knowledge of the exact thickness in this regime is unnecessary. It is important to demonstrate that these metrics are indeed independent of each other. We do this by analyzing dispersions prepared in a way which allows thickness and length to be varied independently. Such analysis ( Supplementary Note 3 ; Supplementary Figs 25 and 26 ) shows that Ext B /Ext 345 and λ A are not intrinsically linked (although there may be a relationship between mean nanosheet thickness and length, which is due to the exfoliation mechanism, see below). In addition, we have shown ( Supplementary Fig. 27 ) that the metrics work well even at the highest dispersion concentrations. This is an important result, which makes it possible to determine both mean length and number of layers for solution-processed MoS 2 nanosheets using two metrics extracted from a simple extinction spectrum, which is measureable in any laboratory. Applying length and thickness metrics We can use these metrics to assess the dimensions of flakes in a wide range of dispersions produced under a range of conditions including simple homogenous centrifugation at different rates as well as samples that were fractionated by BS. Shown in Fig. 5a , is a graph of extinction ratio Ext B /Ext 345 plotted versus λ A for >50 dispersions. It is clear that these data all fall on the same master curve. We can use equations (5 and 6) to transform Fig. 5a into a graph of L versus N ( Fig. 5b ). This curve is interesting, showing a clear correlation between lateral size and thickness. This is not because the metrics are correlated. Rather, it is due to the greater interlayer binding energy associated with larger flakes: they are harder to exfoliate and so are thicker on average. Such a correlation has previously been observed for liquid-exfoliated MoO 3 nanosheets [33] and confirmed in this work on flake by flake measurements of MoS 2 -sodium cholate (SC) ( Supplementary Fig. 28 ). Importantly, Fig. 5b shows that dispersions can be produced with mean values of N close to 1. 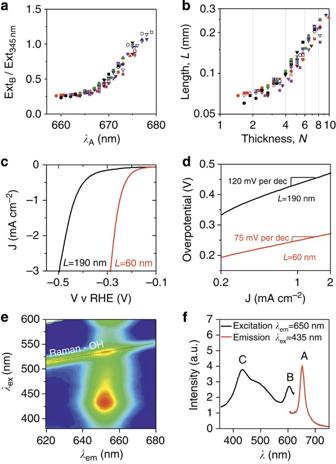Figure 5: Use of the metric for applications and fundamental studies. (a,b) Map of extinction metrics for length and thickness for a number of fractions obtained by band sedimentation under varying centrifugation conditions from various stock dispersions. (a) Raw data from extinction spectroscopy and (b) converted to actual mean length and thickness by using the calibration equations obtained from spectroscopy and microscopy. (c) Linear sweep voltammograms (5 mV s−1) for films of length-selected MoS2on indium tin oxide (ITO) substrates, comparing the electrocatalytic response towards hydrogen-evolution reaction. Measured potentials were subjected to iR correction (see Supplementary Information). Supporting electrolyte was 0.5 M H2SO4. (d) Overpotential versus current density plots showing Tafel slopes expressed as mV per decade (mV per dec). (e) Photoluminescence excitation contour plot of a monolayer-rich MoS2-SC dispersion showing the expected A-exciton fluorescence at 651 nm. (f) Excitation spectrum of the emission signal collected at 650 nm and emission spectrum excited at 435 nm. A, B and C-excitonic features are clearly identified. The Raman signal of O–H was subtracted from the excitation spectrum. Figure 5: Use of the metric for applications and fundamental studies. ( a , b ) Map of extinction metrics for length and thickness for a number of fractions obtained by band sedimentation under varying centrifugation conditions from various stock dispersions. ( a ) Raw data from extinction spectroscopy and ( b ) converted to actual mean length and thickness by using the calibration equations obtained from spectroscopy and microscopy. ( c ) Linear sweep voltammograms (5 mV s −1 ) for films of length-selected MoS 2 on indium tin oxide (ITO) substrates, comparing the electrocatalytic response towards hydrogen-evolution reaction. Measured potentials were subjected to iR correction (see Supplementary Information). Supporting electrolyte was 0.5 M H 2 SO 4 . ( d ) Overpotential versus current density plots showing Tafel slopes expressed as mV per decade (mV per dec). ( e ) Photoluminescence excitation contour plot of a monolayer-rich MoS 2 -SC dispersion showing the expected A-exciton fluorescence at 651 nm. ( f ) Excitation spectrum of the emission signal collected at 650 nm and emission spectrum excited at 435 nm. A, B and C-excitonic features are clearly identified. The Raman signal of O–H was subtracted from the excitation spectrum. Full size image The ability to both control and easily measure nanosheet size and thickness will be extremely useful, facilitating the processing of materials for both applications and basic research. We demonstrate the application of these techniques in both of these areas. First, we demonstrate the utility of accurate size control and measurement by preparing hydrogen-evolution catalysts from solution-exfoliated MoS 2 . The sites responsible for the catalysis of hydrogen evolution by MoS 2 are known to reside on the flake edges [55] , making small flakes desirable and illustrating the need for size control. We prepared two dispersions using distinct centrifugation protocols. The measured extinction spectra were used to determine the mean lateral size of nanosheets (190 and 60 nm) as well as the concentration of dispersed material. Vacuum filtration was used to produce thin films (30 μg cm −2 ), which were transferred onto indium tin oxide-coated glass substrates and characterized for hydrogen-evolution catalysis (see methods and Supplementary Note 1 ). A clear size effect is seen ( Fig. 5c,d ), with considerably lower onset potential and Tafel slope [55] observed for the smaller flakes compared with larger ones. This demonstrates the potential of our method to facilitate optimized sample preparation for applications of nanosheets. Furthermore, the ability to produce dispersions with controlled nanosheet dimensions allows the preparation of samples for more fundamental studies. To demonstrate this, we used size selection coupled with analysis via the thickness metric to produce monolayer-rich (that is, with low average N) MoS 2 dispersions, which allow the study of solution-phase PL. Shown in Fig. 5e is a PL-excitation contour plot for such a dispersion, which shows the direct band gap luminescence associated with monolayer MoS 2 ( λ em =651 nm). The emission spectrum ( λ ex =435 nm) shows a narrow peak (full-width half-maximum=23 nm) that can be fitted to a single Lorentzian, consistent with PL from monolayered MoS 2 . The PL spectrum is size independent with no apparent edge effect other than reduction of PL intensity for very small nanosheets ( Supplementary Note 4 and Supplementary Figs 29 and 30 ). Fluorescence from few and multi-layered species in the dispersion (with a mean thickness of two layers) cannot be resolved due to the significantly lower quantum efficiency [51] . The excitation spectrum (after subtraction of Raman mode of water, λ ex =651 nm) is depicted in Fig. 5f , clearly revealing signatures of the B and C-excitonic transitions. We note that while the measurement of contour maps and excitation spectra is virtually impossible using micromechanically cleaved MoS 2 , it is straightforward in liquid once size selection and measurement techniques are known. Extension of metrics to other nanosheet types The nanosheet extinction metrics described in this paper rely on fundamental principles that both flake edge and degree of exfoliation influence the electronic structure. This implies that this is a general method that can be used for a wide range of liquid-exfoliated nanosheets. To demonstrate this, we show the same changes to extinction spectra for band-sedimented, surfactant-exfoliated dispersions of WS 2 ( Fig. 6 ), MoSe 2 and WSe 2 ( Supplementary Figs 32–33 ). Almost identical behaviour is observed in all materials although the extinction ratio must be calculated using appropriate wavelengths: for WS 2 , we use Ext A /Ext 295 , where A represents the A-exciton position (for example, Fig. 6a–c ). The ability to identify well-exfoliated WS 2 allowed us to prepare dispersions containing very thin nanosheets (that is, with low λ A ). A combination of Raman and PL spectroscopy, coupled with AFM ( Fig. 6d–g ) confirmed such dispersions to be rich in monolayers. Compared with MoS 2 , the WS 2 PL (normalized to the Raman 2LA and nearby modes in Fig. 6h ) appears significantly enhanced. In addition, unlike MoS 2 , the PL associated with WS 2 edges was red shifted and more intense than that from the nanosheet centre ( Fig. 6h ). This suggests that the band gap of the edge region in liquid-exfoliated WS 2 is smaller than that of the centre, in agreement with previous results [56] . Most importantly, neither very small (~50 nm), nor reasonably sized (~300 nm) few-layer species show a notable PL signal further supporting that the nanosheets with a nominal AFM height of 3 nm are monolayered nanosheets. 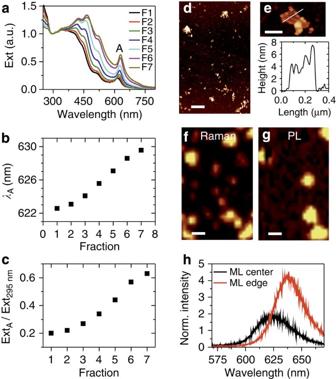Figure 6: Metric for WS2. (a) Extinction spectra, normalized to 295 nm, of surfactant exfoliated WS2fractions after band sedimentation at 2.5k r.p.m. for 10 min. The A-exciton is labelled. (b) A-exciton wavelength plotted as a function of fraction number. (c) Extinction peak ratio, ExtA/Ext295, plotted versus fraction number. (d) Typical AFM images of deposited WS2nanosheets (scale bar, 1 μm) and (e) height profile of the nanosheet at the top right (scale bar, 250 nm). (f) Raman and (g) PL intensity map (532 nm excitation) of the same area (scale bar, 1 μm). (h) Representative PL spectra of the nanosheet displayed ineat the centre and in the edge region. Figure 6: Metric for WS 2 . ( a ) Extinction spectra, normalized to 295 nm, of surfactant exfoliated WS 2 fractions after band sedimentation at 2.5k r.p.m. for 10 min. The A-exciton is labelled. ( b ) A-exciton wavelength plotted as a function of fraction number. ( c ) Extinction peak ratio, Ext A /Ext 295 , plotted versus fraction number. ( d ) Typical AFM images of deposited WS 2 nanosheets (scale bar, 1 μm) and ( e ) height profile of the nanosheet at the top right (scale bar, 250 nm). ( f ) Raman and ( g ) PL intensity map (532 nm excitation) of the same area (scale bar, 1 μm). ( h ) Representative PL spectra of the nanosheet displayed in e at the centre and in the edge region. Full size image In conclusion, we have introduced a simple and versatile centrifugation technique based on BS to rapidly sort liquid-suspended TMDs according to their mass using a normal benchtop centrifuge. This process gave a range of fractions, which had significantly different extinction spectra. Specifically, both the energy of the A-exciton and the relative intensity of the B-excitonic transition varied systematically with fraction number (that is, with nanosheet size). These parameters are related to nanosheet thickness and lateral size, respectively. Statistical measurements of nanosheet length and thickness, made using TEM and AFM, allowed us to quantify these relationships. Such quantification gives access to the determination of mean flake length and thickness in one single extinction measurement. In addition, we find the extinction coefficient at 345 nm to be widely independent of nanosheet thickness and length, allowing the extinction spectrum to be used to measure concentration. The variations in the MoS 2 absorbance and extinction spectra with nanosheet size described above are due to the effects of both confinement and nanosheet edges on the electronic structure of the material. Since these phenomena are general to all 2D materials, the extinction metrics described here can be applied to a range of nanosheet types as we demonstrate for WS 2 , WSe 2 and MoSe 2 . We believe this to be an important result for a number of reasons. On the one hand, the availability of a simple spectroscopic method to measure both thickness and lateral size will be extremely important and will greatly simplify the basic characterization of dispersions of liquid-exfoliated nanosheets. In addition, these results will facilitate the preparation of liquid-suspended nanosheets with well-defined length and thickness distributions. This will be extremely important for applications where nanosheet size is crucial, as well as for understanding fundamental physical properties of layered inorganic materials as a function of size (for example, by fluorescence spectroscopy in solution). Furthermore, this work highlights the influence the edge has on the electronic and optical properties of the nanosheet as a whole. Sample preparation Details are presented in the Supplementary Methods. In brief, TMD dispersions (100 ml) were prepared by probe sonicating (Sonics VX-750) the powder (Sigma Aldrich, typical 20 g l −1 ) in an aqueous SC with the constant weight ratio of SC/TMD=0.3. The resultant raw dispersion was left to settle overnight and subjected to a pre-centrifugation step (Hettich Mikro 220R centrifuge, fixed angle rotor 1016, 750 r.p.m., 60 g ) to remove unexfoliated material. Prior to BS, 1 ml of the stock dispersion of the nanomaterial in aqueous SC was layered on top of the race layer containing 5 ml of deuterated water at the bottom and 5 ml of 1:1 mixture of deuterated water and water (equal surfactant concentrations). After centrifugation in a Heraeus Megafuge 16 benchtop centrifuge equipped with a 3,655 swinging bucket rotor, typically (unless otherwise noted) at 5k r.p.m. (4,695 g ) for 10 min, the seven fractions were collected from the initial 11 ml liquid from top to bottom to obtain samples with standard size and thickness distributions. To obtain larger flakes, conditions were modified: large and thick flakes were enriched in a dispersion by first centrifuging the stock dispersion at 1k r.p.m. (107 g, Hettich Mikro 220R centrifuge, fixed angle rotor 1016). The supernatant was then subjected to a second centrifugation at 2k r.p.m. (425 g ). The sediment after this centrifugation was collected for BS at 2k r.p.m. for 10 min (1,135 g ). To obtain the monolayer-rich dispersion for PLE measurements, the stock dispersion was centrifuged at 5k r.p.m. (2,663 g, 2 h, Hettich Mikro 220R centrifuge, fixed angle rotor 1016), the sediment was discarded, the supernatant was again centrifuged at 15k r.p.m. (22,500 g, 2 h, Hettich Mikro 220R centrifuge, fixed angle rotor 1195-A). After the second centrifugation step, the sediment was reagitated in 0.1 mg ml −1 SC (reducing the initial volume by 50% to yield a high concentration) and subjected to PL measurements. For XPS and electrochemical measurements, the dispersions were vacuum-filtered using porous cellulose filter membranes. For Raman, PL and AFM, dispersions were drop-casted on Si/SiO 2 wafers. Characterization Optical extinction was measured on a Varian Cary 5,000 in quartz cuvettes with a pathlength of 0.4 cm. To distinguish between contributions from scattering and absorbance to the extinction spectra, dispersions were measured in an integrating sphere using a home-built sample holder to place the cuvette in the centre of the sphere of a Perkin Elmer Lamda 650 spectrometer (NB cuvettes need to be transparent to all sides). The absorbance spectrum is obtained from the measurement inside the sphere. A second measurement on each dispersion was performed outside the sphere to obtain the extinction spectrum. This allows calculation of the scattering spectrum (extinction-absorbance). Bright field TEM imaging was performed using a JEOL 2100, operated at 200 kV, while high-resolution TEM was conducted on a FEI Titan TEM (300 kV) on holey carbon grids (400 mesh). Tapping-mode AFM was carried out on a Veeco Nanoscope-IIIa system (Digital Instruments). Raman and PL spectroscopy on substrate was performed using a WITec alpha 300 with 532 nm excitation laser in air under ambient conditions. The PL in solution was acquired on a Fluorolog-3 spectrometer (Horiba Scientific) with a thermoelectrically cooled R928P photomultiplier tube detector. The samples were excited with a 450 W Xe lamp with a double monochromator in excitation (600 grooves per mm, 500 nm blaze grating). XPS was performed under ultra-high vacuum conditions (<5 × 10 −10 mbar), using monochromated Al Kα X-rays (1,486.6 eV) from an Omicron XM1000 MkII X-ray source and an Omicron EA125 energy analyzer. An Omicron CN10 electron flood gun was used for charge compensation and the binding energy scale was referenced to the adventitious carbon 1s core level at 284.8 eV. Mo 3d and S 2p core-level regions were recorded at an analyzer pass energy of 15 eV and with slit widths of 6 mm (entry) and 3 mm x 10 mm (exit), resulting in an instrumental resolution of 0.48 eV. After subtraction of a Shirley background, the core-level spectra were fitted with Gaussian-Lorentzian line shapes and using Marquardt’s algorithm. STEM imaging and STEM-EELS investigations were carried out using an FEI Titan 60–300 Ultimate microscope (‘PICO’) operated at 80 keV, equipped with a high-brightness electron gun, a Cs probe corrector, and a Gatan Quantum postcolumn energy filter system (Ernst Ruska-Centre Juelich). The suspended MoS 2 flakes were dropped onto lacey carbon-coated copper TEM grids that were then heated up to 120°C overnight under vacuum to minimize contamination of the sample. EELS spectra were acquired with a convergence angle of 24 mrad, a collection angle of ~28 mrad, a dispersion of 0.01 eV/channel and an energy resolution over vacuum of 0.1 eV. STEM-EELS maps were acquired with 0.01 s acquisition time per spectra per pixel. Subsequently, the spectra were aligned and calibrated using the zero-loss peak. Individual spectra (1,152) were summed to obtain each of the spectra shown in Fig. 3l . The spectra shown here are representative of a set of 20 STEM-EELS maps that were acquired over similar regions. For the plot of EELS intensity ratio, I 2.8 eV / I 6.4 eV , in Fig. 3m , spectra in three different regions of interest perpendicular to the flake edge were averaged parallel to the edge. Three sets of EELS maps were analyzed in total: set 1:150 spectra acquired over 4.17 nm × 1 nm (direction perpendicular to the edge of the flake) were summed for each spectrum that was analyzed; set 2:282 spectra acquired over 14.67 nm × 0.47 nm (direction perpendicular to the edge of the flake) were summed for each spectrum that was analyzed; set 3:66 spectra acquired over 8.34 nm × 0.51 nm (direction perpendicular to the edge of the flake) were summed for each spectrum that was analyzed. The spectra were then normalized to the intensity of the zero-loss peak. Subsequently, the ratio at 2.8 eV in the EELS to that at 6.4 eV as a function of distance from the edge was plotted. Electrochemical characterization consisted of linear sweep voltammetry (2mV s −1 ) and electrochemical impedance spectroscopy using a three-electrode electrochemical cell and Gamry Reference 3,000 potentiostat. The measurements were performed in 0.5 M H 2 SO 4 solution using a three-electrode electrochemical cell, with a Ag/AgCl (3 M NaCl) reference electrode and graphite rod counter electrode. How to cite this article: Backes, C. et al. Edge and confinement effects allow in situ measurement of size and thickness of liquid-exfoliated nanosheets. Nat. Commun. 5:4576 doi: 10.1038/ncomms5576 (2014).